Symbiont fidelity and the origin of species in fungus-growing ants A major problem in evolutionary biology is explaining the success of mutualism. Solving this problem requires understanding the level of fidelity between interacting partners. Recent studies have proposed that fungus-growing ants and their fungal cultivars are the products of 'diffuse' coevolution, in which single ant and fungal species are not exclusive to one another. Here we show for ants and associated fungi in the Cyphomyrmex wheeleri species group that each ant species has been exclusively associated with a single fungal cultivar 'species' for millions of years, even though alternative cultivars are readily available, and that rare shifts to new cultivars are associated with ant speciation. Such long-term partner fidelity may have facilitated 'tight' ant–fungus coevolution, and shifts to new fungal cultivars may have had a role in the origin of new ant species. Mutualisms occur at all biological levels—from mitochondria within eukaryotic cells to a myriad of species interactions—and they contribute significantly towards increasing complexity in the evolution of life [1] , [2] , [3] , [4] , [5] . The long-term stability and success of mutualisms present a challenge for evolutionary theory, for how can such cooperative associations persist, much less proliferate, when selection favours selfishness and conflict [4] , [6] , [7] ? Answering this fundamental question requires understanding of the level of fidelity between interacting partners. Mutualists can be tightly integrated, resulting in coadaptation and cospeciation (that is, speciation in one partner results in simultaneous speciation in the other), or 'diffusely' associated because of frequent host switching. Diffuse coevolution has been proposed to occur in a variety of mutualisms, such as those between figs and fig-wasp pollinators [4] , [8] , [9] , squids and their bioluminescent bacterial symbionts [10] , and fungus-growing insects and their cultivated fungi [11] , [12] , [13] , [14] , [15] , [16] , [17] . All of the 235 described species of fungus-growing ants (tribe Attini) obligately depend on the cultivation of fungus for food [18] . In return, the ants nourish, protect and disperse their fungal cultivars [18] . Although all attine ants are obligate symbionts, the cultivated fungi vary from facultative to obligate in their associations with ants. In 'lower' attine fungiculture, the ancestral fungicultural system for attine ants [12] , [19] , [20] , fungal cultivars belong to two distinct, separate lineages ('Clade 1' and 'Clade 2') within the tribe Leucocoprineae. Lower-attine fungi are thought to facultatively associate with ants because the fungi can also live outside the symbiosis [12] , [21] . In 'higher' attine fungiculture, however, a highly derived group of fungi descended from a lower-attine fungal ancestor is obligately associated with ants and, as far as is known, cannot live outside the symbiosis [13] , [14] , [16] , [17] , [22] , [23] . Because cultivar clones are typically propagated vertically from parent to offspring nests via transport by foundress queens, it had been long assumed that the two mutualistic partners evolve by strict coevolution (that is, a fungal species evolves in close association with its host ant species) [19] , [24] . However, empirical work over the past two decades has shown that cultivars are frequently transmitted horizontally between different ant colonies (sometimes between colonies of different ant species) and that lower-attine cultivars are closely related to, and in some cases identical to, free-living fungal species, suggesting frequent import of fungi into the symbiosis from free-living sources [12] , [13] , [14] , [17] , [21] , [23] , [25] , [26] , [27] , [28] , [29] . This apparent absence of one-to-one host fidelity (that is, long-term association of ant and fungal genotypes), combined with the recent discovery that the lower-attine fungal Clade 2 ( Fig. 1 ) may be evolutionarily much younger than its ant hosts [16] , has led to a general expectation of low partner fidelity (that is, frequent reassociation of ant and fungal genotypes) in lower-attine fungiculture. 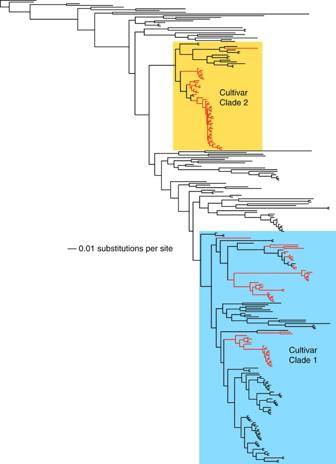Figure 1: Global phylogeny of the fungal tribe Leucocoprineae. The phylogeny was generated by Bayesian analyses of ITS sequence for 405 taxa (271 unique genotypes). Free-living fungi are indicated by black branches. Ant-associated fungi (red branches) have arisen multiple times and are concentrated in cultivar Clade 1 (shown in blue) and Clade 2 (shown in yellow). Figure 1: Global phylogeny of the fungal tribe Leucocoprineae. The phylogeny was generated by Bayesian analyses of ITS sequence for 405 taxa (271 unique genotypes). Free-living fungi are indicated by black branches. Ant-associated fungi (red branches) have arisen multiple times and are concentrated in cultivar Clade 1 (shown in blue) and Clade 2 (shown in yellow). Full size image Because of the difficulty of obtaining large samples of both ants and fungi from the same nests across the full geographic range of a species, most previous work on the fidelity of association of attine ants and their fungi involved reconstructing phylogenies of fungi but not of their ant hosts, or of ants and fungi drawn from limited localities [12] , [14] , [21] , [26] . A complete understanding of the shared evolutionary history of attine ants and their associated fungi, however, requires detailed understanding of the phylogenies of both interacting partners across their geographic ranges [30] , preferably ant–fungus pairs sampled from the same nests. It has long been known that two lower attine species in Panama, Cyphomyrmex longiscapus and C. muelleri , cultivate phylogenetically distantly related fungi from Clades 1 and 2, respectively ( Fig. 1 ), even though nests of the two species occur in sympatry and, indeed, may be separated by only a few centimetres in some localities [12] , [26] , [31] , [32] , [33] . Based on evidence from morphology and biogeography, it was previously hypothesized that C. muelleri may be derived from an ancestor resembling C. longiscapus s.l. and that the origin of C. muelleri may have coincided with, or even have been driven by, a switch from the Clade 1 to Clade 2 cultivar [31] . The younger evolutionary age of Clade 2 relative to Clade 1 [16] is consistent with this scenario, as is experimental work demonstrating that Clade 2-cultivating Panamanian C. muelleri ants accept the cultivar of C. longiscapus , whereas C. longiscapus ants do not readily accept the cultivar of C. muelleri [33] , [34] , reflecting an asymmetric ancestral/derived host-tolerance pattern also known from insect–plant coevolution [35] . These prior observations on the C. longiscapus and C. muelleri symbioses prompted the present investigation of the co-phylogenetic patterns between ants and fungi of these species and their close relatives in the Cyphomyrmex wheeleri group. Here, we reconstruct the relationships of 138 individual ants and 405 fungus-cultivar samples, including ants and fungi taken from the same 88 nests of members of the 'lower' attine C. wheeleri species group (currently consisting of the four species C. wheeleri, C. costatus, C. longiscapus and C. muelleri ) drawn from their known ranges in North, Central and South America. Contrary to expectation, we found that each ant species has been exclusively associated with a single fungal cultivar 'species' for millions of years—even though alternative cultivars are readily available—and that rare shifts to new cultivars are associated with ant speciation. These results strongly support a pattern of ant fidelity to particular fungi in this clade of fungus-growing ants. Global phylogeny of the fungal tribe Leucocoprineae Consistent with previous studies [12] , [21] , our ITS-based phylogeny of the fungal tribe Leucocoprineae ( Fig. 1 ) indicates that associations of fungi with ants have arisen repeatedly, that particular leucocoprineaceous species may be both ant-associated and free-living, and that ant-associated fungi are non-randomly distributed in the phylogeny and concentrated within the 'Clade 1' and 'Clade 2' fungus groups (T-PTP test: n global =271, n Clade 1 =138, n Clade 2 =69; P <0.001). Clade 1 and Clade 2 fungal cultivar phylogenies Within 'Clade 1' and 'Clade 2', cultivar associations with C. wheeleri -group ants are concentrated within particular, narrowly defined lineages ( Fig. 2a and b ). For example, although cultivar clade B ( Fig. 2a ) includes fungi associated with seven observed fungus-growing ant species, a derived lineage within this clade (darker coloured box) accounts for all associations with Cyphomyrmex cf. longiscapus n. sp. 2 and, within this derived lineage, a single genotype (that is, a single ITS sequence-identical strain) (red arrow), occurring in Ecuador, Panama and Costa Rica, accounts for 64 of 70 such associations. Likewise, although cultivar clade D ( Fig. 2a ) includes fungi associated with three observed ant species, a derived lineage within that clade (darker coloured box) accounts for 18 of a total of 20 observed associations with C. longiscapus . Finally, cultivar clade G ( Fig. 2b ) is associated with five observed ant species, but a derived lineage within that clade (darker coloured box) accounts for all observed associations with just two species, C. muelleri and C. cf. costatus sp. 2; within that derived lineage, a single genotype (red arrow), occurring in Ecuador, Panama and Costa Rica, accounts for 49 out of 82 such associations. These patterns indicate that each ant species appears to be exclusively associated with a single species of fungus independent of geography. 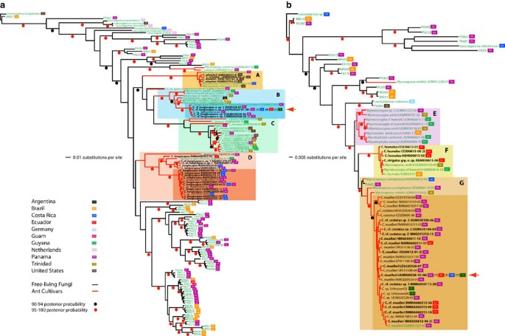Figure 2: Phylogenies of Clade 1 and Clade 2 leucocoprineaceous fungi. (a) Clade 1 and (b) Clade 2. Phylogenies were generated by Bayesian analyses of ITS sequence for 183 and 123 taxa (138 and 69 unique genotypes, respectively). Ant-associated fungi (red branches), designated by associated ant species names and collection IDs, are concentrated in six main clades (A-G, coloured boxes). Within those clades,C. wheelerigroup-associated fungi are concentrated in three sublineages (clades B, D and G) and, within those lineages, exclusively (clades B and G) or largely (clade D) in particular sublineages (darker coloured boxes). Red arrows in clades B and G indicate single widespread genotypes (number of ITS sequence-identical strains indicated in parentheses) that account for the great majority (64 of 70 in clade B; 49 of 82 in clade G) of observed associations. Coloured circles indicate posterior probabilities of clades, and small coloured labels indicate geographic localities (see legend). Fungal sequences listed in black were generated for this study; those listed in green result from prior studies. Figure 2: Phylogenies of Clade 1 and Clade 2 leucocoprineaceous fungi. ( a ) Clade 1 and ( b ) Clade 2. Phylogenies were generated by Bayesian analyses of ITS sequence for 183 and 123 taxa (138 and 69 unique genotypes, respectively). Ant-associated fungi (red branches), designated by associated ant species names and collection IDs, are concentrated in six main clades (A-G, coloured boxes). Within those clades, C. wheeleri group-associated fungi are concentrated in three sublineages (clades B, D and G) and, within those lineages, exclusively (clades B and G) or largely (clade D) in particular sublineages (darker coloured boxes). Red arrows in clades B and G indicate single widespread genotypes (number of ITS sequence-identical strains indicated in parentheses) that account for the great majority (64 of 70 in clade B; 49 of 82 in clade G) of observed associations. Coloured circles indicate posterior probabilities of clades, and small coloured labels indicate geographic localities (see legend). Fungal sequences listed in black were generated for this study; those listed in green result from prior studies. Full size image C. wheeleri group ant phylogeny The ant phylogeny ( Fig. 3 ) indicates that, in addition to four known and two previously hypothesized cryptic species ( C. cf. longiscapus n. sp. 1 and 2 [31] ), currently circumscribed ant species consist of additional, previously undetected, sibling species. C. wheeleri and C. muelleri are each divided into two distinct geographic species, Texas versus California (K2P-corrected distance=0.11) and Ecuador versus Panama (K2P-corrected distance=0.06), respectively. The geographic species pairs in both C. wheeleri and C. muelleri are old, diverging approximately 5.3 and 5.8 mya, respectively ( Fig. 3 ). C. costatus is also divided into two distinct species-level lineages (K2P-corrected distance=0.10) that diverged approximately 7 mya and that co-occur in Ecuador. C. cf. longiscapus n. sp.1, C. cf. longiscapus n. sp. 2, and C. longiscapus co-occur in Panama. 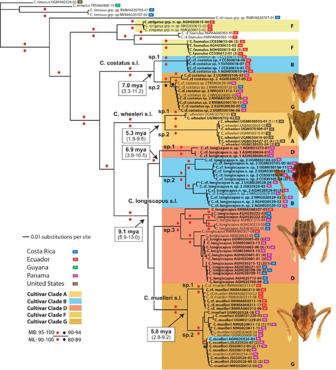Figure 3: Phylogeny of theC. wheelerigroup of fungus-growing ants and outgroup species. The phylogeny was generated by Bayesian (shown) and maximum-likelihood analyses of 1,043 bp of mtCOI and 634 bp of nuclear wingless genes from 138 taxa (96 unique genotypes). Large coloured boxes indicate ancestral associations of ants with the cultivar clades shown inFig. 2, as reconstructed in BayesTraits (all posterior probabilities ≥0.98). Although geographic speciation events withinC. wheeleris.l. andC. muelleris.l. were not associated with shifts in cultivar association, five observed shifts in cultivar association were consistently associated with ant speciation events, for example, inC. costatuss.l. (sp. 1 versus sp. 2),C. longiscapuss.l. (sp. 1 and sp. 3 versus sp. 2) and at the origin ofC.muelleri(C.muelleris.l. versusC.longiscapuss.l.). Divergence-date estimates from Bayesian relaxed-clock analyses are indicated for major lineages. Coloured circles indicate Bayesian posterior probabilities (above branch) and maximum likelihood bootstrap proportions (below branch); small coloured labels beside taxon names indicate localities; numbers in parentheses refer to the number of samples belonging to a given ant genotype; and names in non-bold type indicate ant species for which fungal cultivars were not available. Ant heads from top to bottom:C. cf. costatussp. 2,C. wheelerisp. 2,C. cf. longiscapussp. 2,C. longiscapussp. 3 (syntype specimen) andC. muellerisp. 2. Figure 3: Phylogeny of the C. wheeleri group of fungus-growing ants and outgroup species. The phylogeny was generated by Bayesian (shown) and maximum-likelihood analyses of 1,043 bp of mtCOI and 634 bp of nuclear wingless genes from 138 taxa (96 unique genotypes). Large coloured boxes indicate ancestral associations of ants with the cultivar clades shown in Fig. 2 , as reconstructed in BayesTraits (all posterior probabilities ≥0.98). Although geographic speciation events within C. wheeleri s.l. and C. muelleri s.l. were not associated with shifts in cultivar association, five observed shifts in cultivar association were consistently associated with ant speciation events, for example, in C. costatus s.l. (sp. 1 versus sp. 2), C. longiscapus s.l. (sp. 1 and sp. 3 versus sp. 2) and at the origin of C . muelleri ( C . muelleri s.l. versus C . longiscapus s.l.). Divergence-date estimates from Bayesian relaxed-clock analyses are indicated for major lineages. Coloured circles indicate Bayesian posterior probabilities (above branch) and maximum likelihood bootstrap proportions (below branch); small coloured labels beside taxon names indicate localities; numbers in parentheses refer to the number of samples belonging to a given ant genotype; and names in non-bold type indicate ant species for which fungal cultivars were not available. Ant heads from top to bottom: C. cf. costatus sp. 2, C. wheeleri sp. 2, C. cf. longiscapus sp. 2, C. longiscapus sp. 3 (syntype specimen) and C. muelleri sp. 2. Full size image Contrary to expectation, since their origins, all C. wheeleri group ant species have been tightly associated with narrowly defined fungal groups ( Fig. 3 ) (BayesTraits ancestral-state posterior probabilities [PP] ≥0.98). C. cf. costatus sp. 1, occurring in Ecuador, is entirely associated with cultivar clade B, whereas C. cf. costatus sp. 2, occurring in Ecuador, Costa Rica and Panama, is entirely associated with cultivar clade G. C. cf. longiscapus n. sp. 1 is associated with cultivar clade D, C. cf. longiscapus n. sp. 2 is associated with fungal cultivar clade B, C. longiscapus is associated with cultivar clade D and both C. wheeleri sp. 1 and sp. 2 are associated with cultivar clade A. With a single exception ( C. muelleri sp. 2 AGH020526-03), both C. muelleri sp. 1 and sp. 2 are associated with cultivar clade G. Data on the exception, C. muelleri sp. 2 AGH020526-03, were included in BayesTraits ancestral-state analyses and in ParaFit analyses of coevolution and did not alter the respective conclusions that the ancestor of C. muelleri s.l. cultivated a clade G fungus (PP=1.0) and that significant ant–fungus coevolution has occurred between clade G fungi and their associated ants ( P <0.05). In short, although not all observed ant speciation events are associated with shifts in cultivar association, every observed shift in cultivar association is associated with an ant speciation event. Taken together, these results strongly support a pattern of ant fidelity to particular fungi that is independent of geography and stable over evolutionary time spans of several millions of years. For example, C. wheeleri s.l. consists of two distinct geographic species that have both remained associated with cultivar clade A for approximately 5 million years. Likewise, C. muelleri s.l. includes two distinct cryptic sibling species that have both been associated with cultivar clade G for approximately 6 million years ( Fig. 3 ). Whereas these examples represent cases in which ant lineages have diverged while remaining faithful to the same cultivar, observed shifts to new fungal cultivars have invariably been associated with ant speciation [1] , as discussed above. For example, C. cf. costatus sp. 1 is associated with cultivar clade B, whereas its sister species is associated with cultivar clade G ( Fig. 3 ), representing a shift not only between fungal species but also between Clade 1 and Clade 2 fungi that occurred approximately 7 million years ago. Additional cultivar shifts correlated with ant-speciation events occurred at the origins of C. wheeleri s.l., C. cf. longiscapus n. sp. 1, C. cf. longiscapus n. sp. 2, C. longiscapus and C. muelleri, all occurring 5.3 to 6.9 million years ago. Although this pattern is consistent with a prior hypothesis that shifts in fungal cultivar association may have driven speciation in ants of the C. wheeleri group [31] , it is also consistent with alternative hypotheses, including those in which ant speciation preceded cultivar shifts. It should also be noted that even though the combined nuclear and mitochondrial K2P-corrected distances between C. wheeleri sp. 1 and 2 and C. muelleri sp. 1 and 2 are quite large, it remains possible that one or both of these two purely geographic, non-sympatric species pairs are the highly divergent endpoints of conspecific population clines. This alternative, however, only strengthens our results because, under that scenario, every case of speciation in the C. wheeleri group is then correlated with an ancestral shift in cultivar association. This historical pattern of long-term ant-fungus fidelity for several million years provides the opportunity for coevolution, in which evolutionary modification in an ant host can prompt modification in its fungal symbiont, and vice versa . Because cultivar lineages are associated with multiple ant species, the C. wheeleri -group ant–fungus mutualism cannot be characterized as strict 'one-to-one' coevolution, but neither can it be characterized as broadly diffuse, 'one-to-many,' coevolution. Instead, it might best be characterized as narrowly diffuse, 'one-to-few' coevolution. The C. wheeleri ant clade is closely related to the higher Attini [20] , which includes the leaf-cutting ants whose fungal cultivars are highly derived, obligate symbionts that exhibit coevolved modifications [16] , [20] , [22] . If C. wheeleri -group ant–fungus associations are more specific than those found in other lower Attini, they may represent an intermediate condition linking the broadly diffuse associations found in other lower-attine ants with the narrow associations that led to the evolution of higher-attine fungiculture. Samples and DNA preparation We conducted phylogenetic analyses of C. wheeleri group ants and their associated fungi based on DNA sequence data obtained from a total of 138 ant and 193 fungal samples from Panama, Ecuador, Costa Rica and the United States ( Supplementary Table S1 ). Our data included a subset of 88 nests that yielded exemplars of both ants and fungi. For fungi, we combined 193 fungal DNA sequences obtained for this study with 212 fungal DNA sequences from prior studies [12] , [21] to construct a global phylogeny of 405 leucocoprineacous fungi (reduced to 271 when all but one exemplar of each group of redundant genotypes were excluded; Supplementary Table S2 ). These samples were in most cases preserved in ethanol in the field; some fungi were cultured from gardens of laboratory nests and their mycelium was lyophilized and preserved at −80 °C for later study. Ant vouchers and fungal samples are deposited in the USNM Department of Entomology collections. Information detailing extraction, PCR and sequencing methods can be found in the Supplementary Methods . Alignments and data matrices Ants: For this study we generated sequence data for 138 individual ants consisting of a 1,043-bp COI protein-coding fragment, two wg protein-coding fragments totalling 316 bp and a variable-length wg intron consisting of 220–318 bp. Sequences were edited in Sequencher (Lasergene version 7.0; DNASTAR, Madison, WI) and aligned using ClustalW [36] and by eye. After eliminating all but one representative of each unique genotype and one taxon judged to contain a COI pseudogene, and after excluding 44 bp of autapomorphic indel regions occurring in the wg intron, our ant data set consisted of 96 ant taxa and 1720 nucleotide sites. Because 32 taxa contained one or more missing fragments, for each treatment two phylogenetic analyses were conducted, one with the full 96-taxon data set and one with the 64-taxon data set in which there were no missing fragments. To check for possible gene tree/species tree discordance problems, single-gene analyses were also conducted utilizing data matrices consisting of, for COI, 96 taxa and 1,043 nucleotide characters and, for wg, 68 taxa and 633 nucleotide characters. Fungi: For this study we generated ITS sequence data for 193 ant garden fungi for a variable-length fragment ( ∼ 700–750 bp) of the nuclear ITS region. After eliminating all but one representative of each unique genotype, our fungal data set consisted of 59 exemplar taxa, which we analysed in three separate alignments: global, Clade 1 and Clade 2. Global analyses utilized a data matrix in which the 59 new sequences were combined with 212 leucocoprineaceous sequences generated for previous studies, producing a data matrix of 271 fungal taxa and 721 nucleotide sites. Clade 1 analyses utilized a data matrix of 138 taxa (out of a total of 183 Clade 1 taxa), including all Clade 1 fungi known to be ant-associated, and 838 nucleotide sites. Clade 2 analyses utilized a data matrix of 69 taxa and 950 nucleotide sites. All alignments were produced in the program MAFFT v6.814b [37] using the E-INS-I algorithm, a 200PAM/k=2 scoring matrix, a gap opening penalty of 1.53, and an offset value of zero. Data partitioning Ants: Based on genes and on the variability of codon–position sites within each gene, and based on the results of Ward et al . [38] , we partitioned the ant data set into six partitions: COI first positions, COI second positions, COI third positions, wg first and second positions, wg third positions and the wg intron. Fungi: In global analyses, the fungal ITS region was analysed as a single unpartitioned unit. For Clade 1 and Clade 2 analyses, we partitioned the fungal ITS region into two partitions, a 'rapidly evolving' partition and a 'conserved' partition. In all cases, best-fit models of sequence evolution were selected for each partition under the Akaike information criterion as calculated in ModelTest v3.7 [39] . Bayesian phylogenetic inference All ant and fungal data sets were analysed under Bayesian criteria as implemented in MrBayes v3.1. 2 [40] with nucmodel=4by4 and samplefreq=500 (ants) or 100 (fungi). All parameters, including branch-length rate multipliers, were unlinked across partitions except branch lengths and topology. All analyses were carried out using parallel processing (one chain per CPU) with 8 chains per run and 2 runs per analysis (nruns=2) and consisted of 10 million generations. Maximum likelihood analyses All ant data sets were analysed under maximum likelihood criteria as implemented in Garli 0.97. r737 [41] , [42] using parallel processing. ML bootstrap analyses consisted of 1000 pseudoreplicates, deviating from default settings as follows: genthreshfortopoterm=5000; scorethreshforterm=0.10; startoptprec=0.5; minoptprec=0.01; numberofprecreductions=1; treerejectionthreshold=20.0; topoweight=0.01; brlenweight=0.002. ML 'best tree' analyses consisted of 100 searches, deviating from the default settings as follows: topoweight=0.01; brlenweight=0.002. T-PTP tests The correlation with phylogeny of ant-associated vs. free-living fungi was tested for the global ( n =271), Clade 1 ( n =138), and Clade 2 ( n =69) fungal phylogenies using the T-PTP test [43] with 1000 iterations as implemented in PAUP* v.4.0a118. [44] In each case, the significance of the parsimony-based length difference between the observed tree and the tree in which ant-associated fungi were constrained to be monophyletic was assessed by comparing it to the distribution of such length differences calculated from 1,000 replicates in which ant associations were randomized across fungal taxa. For all three data sets, the observed length difference was consistently less than the length differences for the permuted data, that is, the observed length difference was significant at P< 0.001. Test for coevolution The permutation-based ParaFit test for significant global coevolution between 'parasites' (attine ants) and 'hosts' (leucocoprineaceous fungi) [45] was applied to a reduced data set of 99 ants and 90 fungi, that is, to the largest overlapping subset of ants and fungi for which we had sequence data and host associations and, for ants, for which we had sufficient sequence data to calculate pairwise distances. Distances were calculated for both ants and fungi in PAUP* v.4.0a118 [44] under the GTR+I+G model using maximum-likelihood values for the proportion of sites invariant and gamma alpha calculated in PAUP on maximum-likelihood topologies identified by GARLI-PART 0.97.r737 [41] . Distances were converted into principal coordinate matrices [46] in DistPCoA [47] with negative eigenvalues removed. The principal-coordinate-transformed distance data were analysed in ParaFit using 999 permutations, resulting in significant support for a hypothesis of global coevolution between Cyphomyrmex wheeleri -group ants and their fungal cultivars ( P =0.001), as well as for ant-fungus coevolution in fungal clades A, B, D, F and G ( P <0.05) ( Figs 2 and 3 ). Ancestral state reconstruction We inferred the ancestral fungal lineage for each ant species using the Bayesian method [48] implemented by BayesMultiState in the computer package BayesTraits ( www.evolution.rdg.ac.uk ). We coded each fungal lineage within the Cyphomyrmex wheeleri group (cultivars A, B, D, F, G) as a separate state; in cases where the fungal association was unknown for a particular ant specimen, the state was coded as unknown. We estimated Bayesian posterior distributions for each state using MCMC on a set of 1,000 trees selected randomly without replacement from the total set of post-burnin trees obtained from the MrBayes analyses. As suggested in the program manual, exploratory analyses were conducted to determine the appropriate range for hyperpriors and to select a ratedev value that produced an acceptance rate between 20 and 40%. We used hpall (0, 10) and ratedev=20 for the results reported below; alternative distributions and values produced virtually identical results. The MCMC chain was run for 100 million generations with a burnin of 10 million and sampled every 10,000 generations. The following fungal cultivar lineages were reconstructed at the crown-group node for each ant species: C. strigatus group n. sp., cultivar F with PP=0.99; C. faunulus , cultivar F with PP=1.0; C. costatus sp.1, cultivar B with PP=1.0; C. costatus sp.2, cultivar G with PP=1.0; C. wheeleri , cultivar A with PP=0.98; C. longiscapus sp.1, cultivar D with PP=1.0; C. longiscapus sp.2, cultivar B with PP=1.0; C. longiscapus sp.3, cultivar D with PP=1.0; C. muelleri , cultivar G with PP=1.0. Divergence dating Divergence times for ant lineages within the Cyphomyrmex wheeleri group were inferred under a Bayesian framework using BEAST v.1. 6.1 by employing an uncorrelated lognormal-relaxed clock model [49] , [50] . We used the same nucleotide-partitioning scheme and substitution models as detailed above. Substitution models were unlinked and clock and tree models linked among partitions. A Yule speciation process with a random starting tree was used for the tree prior. We assigned a priori age distributions to two nodes. The root node was assigned a lognormal prior of log(mean)=1.6, log (s.d. )=1.0, offset=15 (equivalent to a minimum bound of 15 Ma, median value of 20 Ma and a 95% quantile of 40 Ma) based on the presence of Cyphomyrmex maya and C. taino , both members of the C. rimosus group, in Dominican amber [20] , [51] . The crown group of the C. wheeleri group was also assigned a normal prior of mean=20, s.d.=5 (equivalent to a median of 20 Ma and a 95% confidence interval of 1.8–18.2 Ma) based on prior divergence dates from a largely independent data set [20] . Elimination of this second prior, which is not directly linked to the fossil record, altered resulting ages by less than 1 Ma. MCMC searches were conducted for 100,000,000 generations with the first 20,000,000 generations discarded as burn-in. Trees and other parameter values were saved every 10,000 generations. Convergence and stationarity were assessed with Tracer v.1.5 [52] using ESS scores, log likelihood values and the consistency of results between multiple runs. The results from two independent runs were combined and visualized using FIGTREE v.1.3.1 [53] . Accession codes : The sequence data have been deposited in GenBank NCBI database under accession codes JQ617314 to JQ617746 listed in Supplementary Tables S1 and S2. How to cite this article: Mehdiabadi, N. J. et al . Symbiont fidelity and the origin of species in fungus-growing ants. Nat. Commun. 3:840 doi: 10.1038/ncomms1844 (2012).